A random forest approach to capture genetic effects in the presence of population structure The accurate mapping of causal variants in genome-wide association studies requires the consideration of both, confounding factors (for example, population structure) and nonlinear interactions between individual genetic variants. Here, we propose a method termed ‘mixed random forest’ that simultaneously accounts for population structure and captures nonlinear genetic effects. We test the model in simulation experiments and show that the mixed random forest approach improves detection power compared with established approaches. In an application to data from an outbred mouse population, we find that mixed random forest identifies associations that are more consistent with prior knowledge than competing methods. Further, our approach allows predicting phenotypes from genotypes with greater accuracy than any of the other methods that we tested. Our results show that approaches that simultaneously account for both, confounding due to population structure and epistatic interactions, are important to fully explain the heritable component of complex quantitative traits. Quantitative trait locus mapping is a powerful approach to study the genetic make-up of diverse quantitative traits, ranging from molecular readouts to organismal phenotypes. One of the most widely used approaches for the analysis of genotype to phenotype relations are linear mixed models (LMMs), which have proven to be reliable and robust in a wide range of genetic designs. A major advantage of LMMs compared with alternative methods is their ability to effectively account for unwanted correlation between samples, thereby correcting for confounding factors such as population structure [1] , [2] , [3] , [4] , [5] , [6] , [7] or hidden covariates [8] . Consequently, LMMs are a widely applied standard approach to analyse associations between individual loci and phenotypes in genetic analysis of model systems [1] , in animal and plant breeding, for example [5] , [6] , [7] , and, thanks to recent computational speedups, now also in large-scale genome-wide association studies (GWASs) in humans [2] , [3] , [9] . A shortcoming of the standard LMM is, however, that it cannot jointly model genetic effects of multiple loci or markers on the readout. Recent work revealed that such single-locus association models are frequently insufficient to explain the heritable component of complex traits [10] , [11] , [12] . Indeed, quantitative traits that involve both linear additive and epistatic (non-additive) effects appear to be the rule rather than an exception. Examples of such complex traits have been identified in the context of physiological [13] , [14] and molecular [15] traits. One approach to address such polygenic trait architectures are multivariate extensions of LMM, either by including multiple fixed effects in the model [16] , [17] or by aggregating over the effect of multiple loci using additional random effect terms [18] , [19] , [20] . While such multivariate approaches have been shown to be effective for explaining linear additive and polygenic genetic components, they do not address non-additive epistatic effects, which for some traits have been shown to explain a larger proportion of phenotypic variation than additive effects [11] . Alternatively, it is straightforward to construct LMMs to test for pairwise epistasis, considering all possible combinations of two locus models [21] . Such exhaustive approaches, however, are computationally demanding and do not address genetic models with more than two loci or other types of non-additive interactions between multiple alleles. Owing to increasing interest in mapping epistatic effects, several integrative mapping approaches have been developed, most of which build on variants of linear models (LMs) that explicitly include pairwise interaction terms. A particular challenge is the enormous number of statistical tests. To mitigate the burden of multiple testing, it has been proven useful to leverage prior information, such as knowledge about metabolic networks and pathways [22] , [23] . While such an approach can help to reduce the overall number of tests conducted, there is the concern that introducing prior knowledge may result in biases that are difficult to handle [23] . Alternatively, it has been proposed to combine the search for epistasis with the mapping of marginal effects, for example, using greedy forward-selection schemes [24] , [25] or by employing Markov Chain Monte Carlo sampling [26] . In particular, approaches based on random bagging techniques [27] have gained considerable attention. Implementations such as random forest (RF) [28] have been shown to accurately capture epistatic effects [10] , [29] , [30] . However, all of these approaches—including RF—assume that correlations between genotype and phenotype are genuine and, unlike the LMM, do not explicitly correct for population structure or other confounding effects. Thus, there is a lack of mapping methods performing both tasks: correcting for population structure while accounting for epistasis. Here, we present a random bagging approach that provides a simple yet efficient correction for population structure along the lines of LMMs while simultaneously enabling multivariate nonlinear association mapping. We term this approach mixed RF and show that it flexibly combines the advantages of the standard LMM and the RF. Related methods, combining random effect models with regression trees or RF, have recently been proposed in different contexts [31] , [32] . In this work, for the first time, we demonstrate how the combination of an LMM and a RF approach enables identifying complex nonlinear genetic architectures, while accounting for population structure. Importantly, our approach also addresses efficient parameter inference, which is essential for applications to larger data sets. First, we validate the mixed RF in extensive simulation studies, finding that the model is able to markedly increase detection power of genuine genetic signals when compared with a standard RF and alternative LMs across a wide range of genetic architectures. We then map hundreds of individual gene expression levels measured in mice, finding that associations uncovered by mixed RF are in better agreement with known pathway annotations than those detected by other methods. Using the same mouse cohort, we apply mixed RF to the genetic mapping of physiological phenotypes, showing that our method is able to recover complex genetic models, which we validate by improved out-of-sample prediction accuracy. Finally, we apply the mixed RF to four lipid-related traits in human GWAS, where we find that lead associations uncovered by our model are in agreement with results reported in large meta-analyses. Modelling genetic associations with generalized forest models Similar to the standard RF, our approach is based on learning decision trees using genetic markers to partition the phenotype data into groups of minimal variance. Thus, similar to LMs, the mixed RF explains trait variance based on genotype information. However, owing to the repetitive partitioning of data into groups and subgroups of minimal variance, decision tree-based methods are able to capture complex nonlinear relationships between predictors (markers). This is profoundly more general than LMs, which are—without specification of interaction terms—not able to capture epistatic genetic architectures. In addition, Bagging [27] , that is, learning individual trees on bootstrap samples and aggregating these over the resulting ensemble, yields the necessary stability of this approach. The mixed RF extends the standard RF by including an additional random effect term (see Fig. 1 ), which is the same modelling principle that leads to the success of LMMs [17] , [33] , [34] . At every stage of building a mixed forest decision tree, trait variation is modelled by a split according to a selected genetic marker and the random effect. As a consequence of this joint modelling approach, markers tend to be selected that lead to splits minimizing those parts of trait variance that are not captured by the random effect (population structure). The sum over all variances attributed to a given marker (when used for splitting) can then be used as a marker score (see Methods for details). 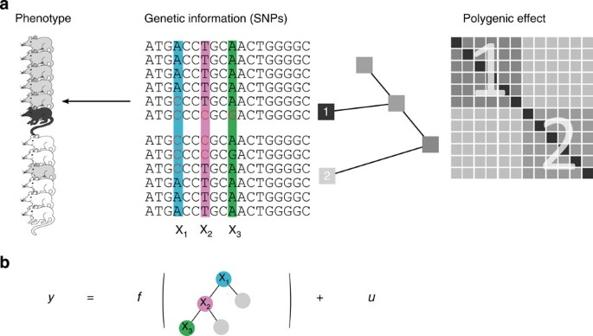Figure 1: Schematic overview of the mixed random forest approach. (a) Individuals are descendants from two different populations as illustrated by the phylogenetic tree. Relatedness between individuals and polygenic effects are captured by the random effect term (covariance matrix, right). Submatrices corresponding to within relatedness of the two populations are indicated by numbers. Remaining parts of the matrix model cross-relatedness. (b) Phenotypes in the population (coat colour) are modelled by the sum of a (genetic) fixed effect and a random effect. The genetic effect is captured using an ensemble of forests; at the same time, the random effectuwith the genetic kinship derived from the population phylogeny explains population structure effects. As a result of this joint learning, splits in the random forest are more likely to occur along informative genetic features that are orthogonal (that is, not correlated) to population structure. In this example, the mouse coat colour is a nonlinear function of the three polymorphic sites X1, X2and X3. Figure 1: Schematic overview of the mixed random forest approach. ( a ) Individuals are descendants from two different populations as illustrated by the phylogenetic tree. Relatedness between individuals and polygenic effects are captured by the random effect term (covariance matrix, right). Submatrices corresponding to within relatedness of the two populations are indicated by numbers. Remaining parts of the matrix model cross-relatedness. ( b ) Phenotypes in the population (coat colour) are modelled by the sum of a (genetic) fixed effect and a random effect. The genetic effect is captured using an ensemble of forests; at the same time, the random effect u with the genetic kinship derived from the population phylogeny explains population structure effects. As a result of this joint learning, splits in the random forest are more likely to occur along informative genetic features that are orthogonal (that is, not correlated) to population structure. In this example, the mouse coat colour is a nonlinear function of the three polymorphic sites X 1 , X 2 and X 3 . Full size image Improved detection of additive and epistatic effects To validate the mixed RF, we initially considered synthetic data sets where the ground truth genetic architecture is known. We used genotype data in the form of 1,000 unlinked single-nucleotide polymorphisms (SNPs) subsampled from 214,553 genome-wide SNPs being part of an Arabidopsis thaliana data set [35] . These data are well suited for this test as the given A. thaliana population is very structured and hence, effects due to population structure can be effectively simulated [35] . To explore a large space of plausible genetic architectures, we considered a total of 20 distinct simulation settings and simulated 50 independent quantitative traits for each. Across the settings considered, we varied the complexity of the trait (that is, number of causal variants), the relative importance of additive and epistatic genetic effects, the magnitude of confounding due to population structure and other parameters (see Methods). We then compared alternative association models and assessed their ability to recover the true causal genetic markers. In addition to the mixed RF, we included a standard RF and the least absolute shrinkage and selection operator (LASSO) in the comparison. Furthermore, we considered a recently proposed extension of the LASSO that, similarly to the mixed RF, accounts for a random effect contribution of population structure. Importantly, the LMM LASSO [17] assumes that genetic effects obey a solely linear additive architecture, as the model does not permit epistatic effects. For reference, we also included standard linear regression (LM) and a LMM, both of which perform independent tests of single loci (see Methods). For each of the 20 simulation settings, we compared the accuracy of the considered methods in terms of the area under the precision–recall curve. Briefly, this approach quantifies the precision (proportion of correct predictions) as a function of the recall (sensitivity), thereby avoiding choosing arbitrary cutoff values for significance when comparing alternative methods (see Supplementary Fig. 1 for an example of a typical precision–recall curve). As expected, the standard RF is more accurate than any of the linear additive models in regimes where epistatic effects dominate the association signals ( Fig. 2a ). However, the performance of RF is severely affected by population structure ( Fig. 2b ). RF is outperformed by LMs correcting for population structure, whenever traits are significantly affected by confounding. Unlike RF, our mixed RF is not affected by such confounding, demonstrating how the proposed random effect extension is able to account for population structure. The mixed RF also performs favourably with respect to the fraction of epistatic interactions ( Fig. 2b ) and the number of causal variants ( Fig. 2c ). Notably, even in the limit of a purely additive architecture ( Fig. 2a ), the mixed RF achieves a level of accuracy similar to that of the LMM LASSO, which a priori imposes a linear additive genetic architecture. 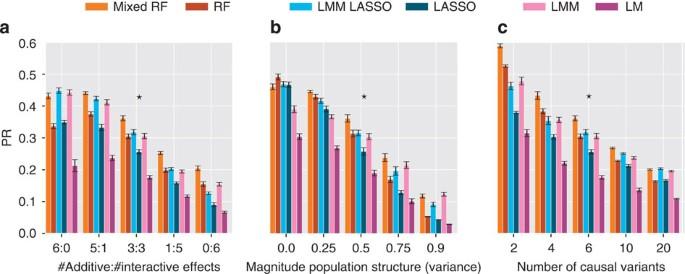Figure 2: Comparison of alternative methods to identify causal genetic loci on alternative simulated data sets. The proposed mixed random forest (mixed RF) is compared with the standard random forest (RF), a univariate linear association test (linear model) and a multivariate linear model (LASSO). We also consider extensions of both linear models to account for polygenic background (LMM and LMM LASSO). Methods are assessed by their ability to recover true causal loci as measured by the area under the precision–recall curve (PR). The baseline setting (as indicated by the asterisk) corresponds to three additive and three multiplicative effects and 50% of the phenotypic variance explained by population structure (seeSupplementary Fig. 1for the PR curves that correspond to this setting). In individual simulations, we altered the ratio between (a) direct additive and epistatic effects, (b) the relative magnitude of population structure (explained variance) and (c) the number of causal genetic variants. Error bars correspond to (empirical) s.e. estimated from five independent restarts of each simulation experiment with different random seeds. Figure 2: Comparison of alternative methods to identify causal genetic loci on alternative simulated data sets. The proposed mixed random forest (mixed RF) is compared with the standard random forest (RF), a univariate linear association test (linear model) and a multivariate linear model (LASSO). We also consider extensions of both linear models to account for polygenic background (LMM and LMM LASSO). Methods are assessed by their ability to recover true causal loci as measured by the area under the precision–recall curve (PR). The baseline setting (as indicated by the asterisk) corresponds to three additive and three multiplicative effects and 50% of the phenotypic variance explained by population structure (see Supplementary Fig. 1 for the PR curves that correspond to this setting). In individual simulations, we altered the ratio between ( a ) direct additive and epistatic effects, ( b ) the relative magnitude of population structure (explained variance) and ( c ) the number of causal genetic variants. Error bars correspond to (empirical) s.e. estimated from five independent restarts of each simulation experiment with different random seeds. Full size image Because the mixed RF combines concepts from LMM and RF, we also considered applying these modelling steps independently using a two-step approach. Supplementary Fig. 2 shows additional results when first fitting the random effect (using the best linear unbiased predictor (BLUP) [36] ) to then apply a standard RF model on the residuals (Methods). This conceptually simpler RF-BLUP model performs considerably worse than the mixed RF, demonstrating the merits of a joint modelling approach. This is in consensus with related work showing that shrinkage, as caused by BLUP, on the first stage of two-stage approaches should be avoided [37] , [38] . Finally, we considered additional simulation settings, where we altered the signal-to-noise ratio, thereby simulating weaker genetic effects ( Supplementary Fig. 2d ), resulting in the same relative ranking of methods. In sum, these experiments give confidence that the mixed RF is a robust tool to identify genotype–phenotype associations in a wide range of settings, addressing both epistasis and population structure. Mixed RF detects functionally consistent associations A significant drawback of simulations is that they inevitably require to make assumptions about the genetic architecture of traits and the nature of noise in the data. We therefore sought to additionally assess mixed RF based on quantitative trait loci (QTL) data without requiring any assumptions about how traits are affected by genetic variants. However, in real settings, accurate ground truth information for genotype–phenotype associations is difficult to obtain and hence it is necessary to revert to a bronze standard. Our approach is based on the notion that expression QTLs (eQTLs) at genes that are functionally related to the target genes whose expression they affect are more likely to be true than eQTLs not fulfilling this criterion [10] . A possible concern of this approach is that several genuine associations may not be in agreement with the pathway databases, for example, because of incomplete annotations or tissue-specific genetic effects. Moreover, in this benchmark we cannot assess the accuracy of cis -eQTLs (that is, when the marker is close to the target gene itself), because the pathway-based analysis only makes sense if two genes (source and target) are involved in an eQTL (see Supplementary Fig. 3 for the relative proportion of cis - and trans -eQTLs detected). Nevertheless, this scheme to assess associations provides a robust test, as results are aggregated over hundreds of target genes and individual eQTLs. We considered gene expression levels from mouse hippocampus as phenotypes [39] and assessed the plausibility of eQTLs using known pathways obtained from the Reactome database [40] . Because of the low number of unique genetic markers (12,545, from an inbred cross of eight founders), we applied each model on a per-chromosome basis where the population structure was estimated from all remaining chromosomes. While this leave-one-out approach may miss inter-chromosomal epistatic interactions between markers, it has been shown to avoid proximal contamination when the same SNPs are used for mapping and for estimating population structure [33] . Analogous analyses when using all genome-wide markers to account for population structure lead to similar overall conclusions where the performance of all mixed-model-based approaches was decreased ( Supplementary Fig. 4 ). Expression traits were selected based on their variance across the population and the genes’ pathway memberships (see Methods for details). This filtering resulted in 300 expression traits considered for the subsequent analysis. Putative causal genes were selected within a 500-kb window around the marker SNPs. A trans -eQTL was termed ‘plausible’ (consistent with the Reactome database) if the respective target gene and any of the genes associated with the marker were annotated as members of the same pathway. Subsequently, we evaluated the QTL mapping methods by ranking the QTLs for all traits jointly based on the respective QTL scores (see Methods). We then compared the observed number of ‘plausible’ associations among the top-scoring eQTLs with the number of expected ‘plausible’ associations if the ranking was random ( Fig. 3 ). 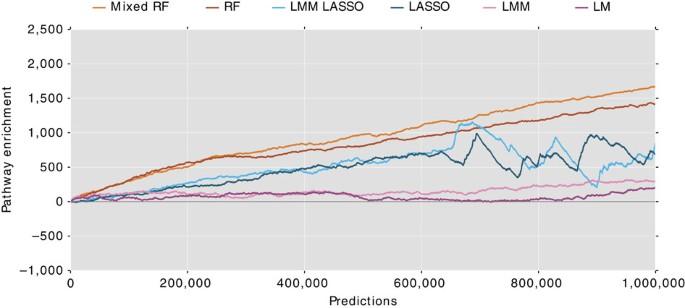Figure 3: Assessment of alternative methods considering Reactome pathway consistency of detected eQTLs on the mouse expression data set. Considered were eQTLs for 300 gene expression traits mapped using the identical methods as considered inFig. 2. We ranked all eQTL scores for all 300 traits together and computed a pathway enrichment score quantifying the number of eQTL–trait associations that are consistent with Reactome (see Methods). The enrichment scores are adjusted for the number of consistent eQTL–trait pairs that are expected for a random ranking. Figure 3: Assessment of alternative methods considering Reactome pathway consistency of detected eQTLs on the mouse expression data set. Considered were eQTLs for 300 gene expression traits mapped using the identical methods as considered in Fig. 2 . We ranked all eQTL scores for all 300 traits together and computed a pathway enrichment score quantifying the number of eQTL–trait associations that are consistent with Reactome (see Methods). The enrichment scores are adjusted for the number of consistent eQTL–trait pairs that are expected for a random ranking. Full size image Notably, all considered methods identified regulator–target gene associations with greater frequency than random assignment, which confirms that this assessment using the Reactome database is an informative criterion to evaluate alternative association methods. Moreover, the systematic difference between linear association models and the RF approaches underlines once more the importance to account for epistatic effects [11] , [30] , [41] . This analysis also confirms that correcting for population structure is important: methods correcting for population structure performed better than their non-correcting counterparts (LMM versus LM; LMM LASSO versus LASSO and mixed RF versus RF). Although this trend was weak, we observed it consistently for all three classes of mapping methods considered. Finally, the proposed mixed RF yielded associations that are more enriched among known pathway annotations than any other method, again demonstrating the merits of combining methods to correct for confounding with non-additive association mapping. The differences between the RF and the mixed RF were strongest in the tail of the association distribution, suggesting that, in particular, weak associations are obscured by population structure, if not accounted for. Mixed RF improves phenotype prediction Complementary to evaluating methods in terms of their ability to recover genuine genetic associations, the ability to predict phenotypic variation from genotype has gained considerable attention, in particular in the field of animal and plant breeding, for example, [42] , [43] , [44] , [45] and also more recently in the genetic analysis of model systems [11] , [46] and human genetics [47] , [48] . Existing approaches to predict phenotype from genotype include dynamical systems approaches to model organism/environment interactions [43] , or employ (regularized) linear regression methods using genome-wide SNP markers [42] , [44] , [48] or random effect models using a kinship matrix [11] , [45] , [46] , [48] . The task of phenotype prediction is also linked to ‘missing heritability’, and several studies have noted that single-marker association methods are not sufficient to fully explain the heritable component of phenotype variability [11] , [12] , [42] , [46] . More complex genetic models, for example, considering epistatic effects, have been shown to significantly improve the fraction of explained phenotypic variance in out-of-sample prediction experiments [11] , [12] . To this end, we also investigated the ability of mixed RF to predict phenotype from genotype. Our assessment is based on 124 phenotypes measured in heterogeneous stock mice [49] , which is the same outbred population of mice considered in the eQTL analysis above. As physiological and behavioural traits are highly complex, we expected them to be affected by a comparably large number of genetic variants. We compared our mixed RF with RF, LASSO and, its counterpart modelling population effects, LMM LASSO [17] . Univariate linear approaches (that is, LMM and LM) were not included in this analysis, as they are conceptually inappropriate for prediction tasks. In addition, we considered BLUP for this prediction task [36] , which is equivalent to mixed RF and LMM LASSO, when the estimation of direct genetic factors is dropped such that prediction is solely based on the (marginal linear) model of the polygenic background. Prediction accuracy of alternative models was assessed using five restarts of a fivefold cross-validation experiment, considering the squared correlation coefficient ( R 2 ) between model predictions and the held-out phenotypic values ( Fig. 4a ). A complete list of the prediction performance of different methods for all phenotpyes is provided in Supplementary Data 1 . To compare the relative prediction performance of different methods, we reported the fraction of phenotypes for which one method outperforms another (requiring that the difference in average R 2 across restarts is greater than the s.e.). Using this approach, we find that mixed RF improves over alternative methods for 58.9% (RF), 55.6% (LMM LASSO) and 57.3% (BLUP) of the phenotypes. Conversely, alternative methods achieve predictions better than mixed RF in only 23.4, 7.3 and 8.1% of all phenotypes (see also Supplementary Fig. 5 for the remaining comparisons). 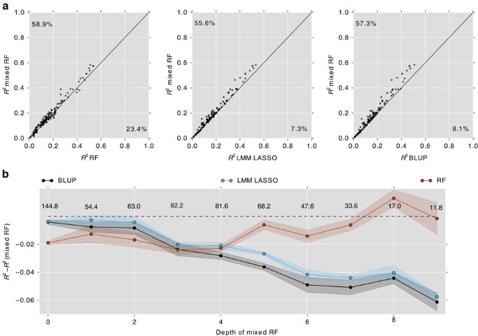Figure 4: Prediction accuracy of mouse phenotypes. (a) Out-of-sample prediction accuracy for alternative methods and for 124 mouse traits is assessed using fivefold cross-validation. Shown is the out-of-sample squared correlation coefficient (R2) for each method and phenotype. Average prediction accuracy and empirical s.e. are estimated from five random restarts. Compared is the mixed RF approach with the standard RF, LMM LASSO and BLUP by correlation plots. (b) Performance of alternative models as a function of trait complexity as estimated by the fitted mixed RF tree depth. For each method, we consider all cross-validation folds fromaand group correlations to held-out samples by the optimal depth found for the corresponding mixed RF. Shown is the average relative prediction accuracy compared with the mixed RF. Shaded areas indicate s.e. estimated (from random restarts). The numbers denote the average number of folds assigned at each given depth. Figure 4: Prediction accuracy of mouse phenotypes. ( a ) Out-of-sample prediction accuracy for alternative methods and for 124 mouse traits is assessed using fivefold cross-validation. Shown is the out-of-sample squared correlation coefficient ( R 2 ) for each method and phenotype. Average prediction accuracy and empirical s.e. are estimated from five random restarts. Compared is the mixed RF approach with the standard RF, LMM LASSO and BLUP by correlation plots. ( b ) Performance of alternative models as a function of trait complexity as estimated by the fitted mixed RF tree depth. For each method, we consider all cross-validation folds from a and group correlations to held-out samples by the optimal depth found for the corresponding mixed RF. Shown is the average relative prediction accuracy compared with the mixed RF. Shaded areas indicate s.e. estimated (from random restarts). The numbers denote the average number of folds assigned at each given depth. Full size image A feature of mixed RF is that it allows us to iteratively increase the depth of the trees in the ensemble, until predictive performance cannot be further improved (see Methods). Whereas, from a practical perspective, fitting this parameter helps to decrease the runtime of our approach, it can also serve as a measure of model (that is, trait) complexity. An ensemble of deep trees (that is, models with many markers) indicates that a given trait is affected by many genetic variants in the respective study population. We used that notion to investigate the performance of mapping methods as a function of trait complexity ( Fig. 4b ): we quantified each trait’s complexity as the depth of the respective mixed RF model and subsequently analysed the performance of the association methods as a function of that measure. Note, as depth was estimated within each of a total of 620 cross-validation folds, some traits may end up in several complexity classes. In general, we observed that the proposed mixed RF is the most robust predictor across the entire spectrum from simple to complex traits ( Fig. 4b ). Whereas linear methods (BLUP and LMM LASSO) perform similarly to mixed RF for simple traits ( Fig. 4b , tree depths ≤2), their predictive power breaks down for more complex traits (that is, tree depth >2). In particular, the improved performance in comparison with the LMM LASSO indicates that a nonlinear structure (such as, epistatic effects) is present in the data, which is better captured by the regression tree-based approaches. Furthermore, RF and mixed RF become similar in performance if the fitted depth of the ensemble gets large ( Fig. 4b , tree depths >4). A possible explanation is that the amount of variance attributable to population structure decreases in relative magnitude as the trait complexity increases and/or that assuming linearity to model population structure is adverse for some of these phenotypes. On this note, we found for tree depths of 8 and 9 (where the standard RF shows best average performance) the (average) number of folds is low (17 and 11.8) when compared with the total of 620 folds considered for each restart of the fivefold cross-validation (indicated by numbers on the top of Fig. 4b ). The small number of folds with tree depth >9 were excluded from this analysis, as they constituted on average less than 10 folds per depth. Application of mixed RF to human GWAS To demonstrate the applicability of mixed RF to human GWAS data, we considered genotype and phenotype data from the Northern Finland Birth Cohort (NFBC) [50] . We applied the mixed RF to four lipid-related traits in a cohort of 5,256 individuals (see Methods for details on preprocessing and analysis). From a total of 328,515 genetic features (SNPs), we report the 40 most associated features identified by the mixed RF. Among these, 29 loci have previously been confirmed in a large meta-study [51] or have been identified using alternative methods applied to the same data [52] (see Supplementary Data 2 ). For this particular mapping experiment, we used an ensemble of 250 trees, where fitting a single tree took on average 13 h and 50 min on a single core (s.d. 3 h and 50 min). The memory usage was below 20 GB (see Methods for further details to the hardware used). Here, we presented an extension to the popular LMMs. By combining the strengths of random effect modelling with tree-based models, our approach is capable of producing robust predictions and phenotype associations over a wide range of potential use cases, and particularly in scenarios where both, polygenic- and nonlinear effects such as epistasis co-occur. We compared the proposed mixed RF to four state-of-the-art methods, each of which have previously been shown to be superior in their respective modelling domain (epistasis, multiple additive and/or polygenic effects) [10] , [17] , [34] , [53] . Results on simulated data showed that mixed RF is not only the most robust across these different domains but also outperforms all competitors when multiple epistatic and polygenic effects are present. On real QTL data from heterogeneous stock mice, we showed that mixed RF recovers more effector–target gene relationships than any of the other methods. Finally, we demonstrated practical scalability to moderately sized GWAS data sets by applying mixed RF to genotype and phenotpye data from the NFBC. Similar to RF, LASSO and LMM LASSO, the proposed mixed RF is capable of modelling more than a single genetic feature at a time, which renders it useful for prediction tasks. On held-out mouse phenotypes, we found that mixed RF is the best predictor for the majority of phenotypes considered. Moreover, it is the only method that is consistently among the top predictors across the entire range of trait complexity. Although mixed RF performs well in a number of settings, the model of course has limitations. First of all, as for any bagging approach, the computational demand is generally larger when compared with alternative (linear) methods. Our implementation of the mixed RF scales linearly with the number of genetic features included in the study, thus having the same runtime complexity as a standard RF. Although our model faces the same limitations as a standard LMM, that is, runtime increases cubical with the number of samples, we note that in analogy to recent speedups for LMMs [2] , computational tricks combined with low-rank approximations to the population structure covariance could be employed to scale the mixed RF to even larger cohort sizes. A second limitation of RF methods is the lack of closed-form statistics to assess the significance of individual markers in the fitted model. Efficient computational strategies to estimate P values and false discovery rates for multivariate models such as the LASSO and RF is an active area of research (see, for example, ref. 54 ). At present, the most robust approach is to estimate empirical P values using permutations [55] . This approach is state of the art for standard RF genetic mapping [30] , [56] , and can be directly adapted to the mixed RF (see discussion in Methods). We also note that simulation-based approaches have been successfully applied to LMMs [57] , [58] and could therefore be an interesting alternative. While our mixed RF adds interpretability to the model by dissecting trait variance into direct genetic and polygenic contributions, interpretation of the RF component remains a challenge. For example, while RF and mixed RF account for epistatic interactions, it is non-trivial to determine which of the markers considered significant are in epistasis with each other (if any). We have recently proposed a method for extracting epistatic interactions from RFs [30] , which is readily applicable to mixed RF. We also note that the objective assessment of the prediction performance when predicting phenotype from genotype needs to be interpreted with care. It is commonly observed that cross-validation accuracies degrade when the extrapolation to fully independent test cohorts is considered (see for instance discussion in ref. 47 ). Nevertheless, cross-validation is valid for the relative comparison of alternative methods. An appealing feature of mixed RF is that model complexity can be flexibly adjusted to the data: since only a subset of samples is used to build each tree, the remaining, so-called ‘out-of-bag samples’ are left over to fit the optimal depth of the trees. This mechanism to control model complexity is implemented into our method and does not require further input by the user. Importantly, the learned tree depth provides insight into the relevance of the fixed genetic effects in relation to the polygenic background—or in other words—this approach can be used to quantify the complexity of the trait. In principle, tree depth can be adjusted for the RF as well. However, its interpretability is limited, because the relative contributions of direct genetic effects and polygenic background to the overall complexity cannot be disentangled. Although it may seem trivial that an optimal model should account for the true number of (genetic) factors contributing to trait variation, there is a scarcity of examples actually performing such model adjustment. Methods such as bagging create an additional computational overhead, which in the past may often not have been deemed necessary. Our results question this view—at least when it comes to explaining trait variation. In the past, the ‘mystery’ of missing heritability has already been attributed to multiple factors. While some of these have been analysed in isolation [11] , [12] , [59] , [60] , our analysis revealed the importance to combine fixed additive effects, epistatic interactions and polygenic effects into a joint model for best explaining the heritability of complex traits. Mixed RF model In the following, we denote y as the response vector of phenotypic observations in N samples, y =( y 1 , …, y N ), and X as the matrix that contains the genetic state of the matching samples at M genetic loci, X =(x 1 , …, x M ). Depending on the genetic system, different encodings for X can be used. For the ease of the following presentation, we assume a binary encoding that can be directly used for homozygous systems, where ‘0’ corresponds to the major allele in the population and ‘1’ denotes the minor allele. However, the proposed method and all derivations can straightforwardly be extended to multiple states such as heterozygous genetic systems. We assume that a phenotypic trait y can be modelled in an additive fashion Here, u denotes a random effect capturing the (polygenic) background and corresponds to independent Gaussian noise. The genetic effect of interest is parametrized by F( X ). In case of a linear relationship F( X )= Xβ , the model implied by equation (2) corresponds to the widely used LMM (for example, refs 1 , 2 , 3 ). Here, it is our goal to fit more general nonlinear relationships with F( X ). We approach this by learning an ensemble of regression trees each grown on a random subsample to infer a noisy variant of the genetic fixed effect. Learned trees reflect the contribution of individual genetic features to the phenotypic variance rather than the global correlation—or family structure, which is captured by the random effect. First, we establish the inference of the genetic fixed effect f t ( X ) for a single regression tree. We then follow the bagging principle as implemented in the standard RF, and our final prediction for F( X ) is computed as the average over the individual fixed effects inferred by the trees. Ordinary regression trees are grown by recursively partitioning the data, such that with each split the reduction in phenotypic variance (Δ R ) is maximized—or equivalently—the sum of the within variances of the resulting partitions R ( t L )+ R ( t R ) is minimized ( t L and t R denote the left and right tree induced by the considered split, respectively). The set of viable splits is determined by the available genetic features. In the case of binary encoding, each feature x j implies exactly one viable split, separating the samples i for which x ij =1 from the ones having x ij =0. We therefore search our space of genetic features to determine index of the feature maximizing the reduction in variance at a given node t , that is, The key insight to derive the mixed RF is to rewrite this splitting criterion (Δ R ) as the corresponding log likelihood of a LM, which has the form: Here, y ( t ) is the vector of observations associated with node t . ( y ( t L ), y ( t R )) T is the reordered version of y ( t ), such that individuals are assigned to the part of the sample with x ( t ) ij =0 ( y ( t L )) and x ( t ) ij =1 ( y ( t R )), respectively. In this representation, β b and β j denote sample bias at node t and splitting weight of x j . denotes the unmodeled residual variance. More concisely we write equation (3) as Using this notation, we can cast the split optimization (equation (3)) in a LM perspective where hats indicate parameters that are estimated using maximum likelihood. In the LM representation, the splitting likelihood in equation (4) can be straightforwardly extended to a LMM accounting for the polygenic background covariance Σ (refs 2 , 9 ) Here, denotes the variance that can be attributed to the polygenic background covariance and we have defined . The new objective for determining the best split is then To maintain tractability of maximum likelihood inference of the model parameters, we utilize the same computational tricks as in refs 2 and 9 (see Supplementary Note 1 for details). Similar to RF, we achieve robustness of our method by learning an ensemble of mixed forest regression trees, each grown on a random subsample of the data. Here, we make the assumption that the effect of population structure on a given bootstrap sample is similar to that of the entire data. To leverage the LM perspective from equation (5), we subset the rows and columns of Σ accordingly, rather than (re)computing the local kinship matrix for each tree. Similarly, we estimate δ on the null model for the entire ensemble, which is analogous to popular approximations in the classical LMM [2] , [9] . To predict the phenotype to a given test genotype x * , we traverse each learned tree in the ordinary decision tree manner until we reach a terminal node and return its associated mean. Analogously to a standard RF, the response m * is computed as the average over the means returned by the individual trees. In addition, population structure captured by the random effect term contributes to the predictive distribution, similar to BLUP [36] . Under the random effect model, the joint distribution of training and test responses is a multivariate Gaussian where the mean is given by the training-fixed effect m as fitted during the forest-building procedure. The training covariance matrix Σ X , X and the cross-covariance are obtained by subsetting Σ , which can be estimated from the whole-genome predictor matrix or selected subset regions (for example, chromosomes; see the Mouse eQTL-mapping experiment). Our prediction for the phenotype of the seen genetic feature x * is the mean of the conditional distribution y * | y , which can be directly derived from the joint distribution (equation (7)) This predictive mean is independent of . Furthermore, we can reuse the δ learned from the null model, and thereby obtain all quantities needed to compute (see also Supplementary Note 1 and ref. 61 for further details). Note that with this model, we choose to infer the fixed effect as an average over individual tree-based fixed effects and make single estimation of the population effect in a separate step. Alternatively, one could consider to estimate both, fixed and population effects for each tree and use the average as a final prediction. In our experience, both approaches yielded near-identical results and we therefore chose the computationally more efficient variant to make a global estimation of the population effect. The optimal tree depth can be efficiently selected while training, where only the training proportion of the data set is used. For each tree t , we use the out-of-bag sample (that is, the part of the training set that was not used building t ) to compute the so-called out-of-bag prediction. We proceed analogously to the ensemble prediction shown in equation (7) with two exceptions. First, the genetic fixed effect is now computed from a single tree alone (instead of the average over the trees), and second, the random effect in this model contains the cross-covariances between in-bag and out-of-bag samples (rather than the cross-covariances between training and test sample). For each tree t , we formalize this model as follows: The estimation of the fixed effect is the vector composed of the tree’s response m o given the out-of-bag sample X o , and the mean fitted for the in-bag sample m b . The (cross)covariances of this model are obtained by subsetting Σ . We can now use the entire tree-based model to make a prediction for , computing the conditional (Gaussian) distribution of . Averaging over all trees up to a particular depth, we obtain the out-of-bag prediction of the whole training vector , which is compared with y by the mean squared error. We (re)evaluate this error after each cycle of the forest-growing procedure increasing the depth of all trees by one. Tree growing is stopped if the error is not decreasing any further. The (forest) depth resulting in the lowest error is used for prediction on the independent test sample. We note that—when using this approach to control for model complexity—care needs to be taken when combining this approach with specific feature importance measures for RFs. For example, the relevances reported by the permutation importance [28] measure may be biased, at least if the same out-of-bag samples are used that determine the tree depth. Implementation details The mixed RF is a python-based implementation providing an interface similar to the learning methods contained in scikit-learn [62] . Core routines that require a significant amount of runtime (such as, the splitting procedure) were implemented in the C++ programming language. For RF, we used the implementation provided by the scikit-learn python package [62] . We adapted the contained RF module [63] to also return the feature scores as used by our method and the random forest R package [64] . Feature importance and statistical significance Following prior work on RFs [10] , we consider the analogue to the residual sums of squares importance measure (RFRSS). On the level of an individual split, the RFRSS can be equally regarded as the log-likelihood ratio of the model considering a split/feature and the alternative that just fits a common mean (see equation (3)). In contrast to the standard RFRSS, we compute the analogue log-likelihood ratio under the LMM (equation (5)). Importantly, RFRSS and our derived score are proportional in the limit of no population structure (when either δ tends to infinity or the estimated kinsip matrix is the identity). While this approach has been shown to be effective for ranking features [10] , it does not directly yield statistical significance levels of individual features. To this end, we note that permutation schemes have been successfully combined with RFs for use in genetics [30] , [56] . These approaches can be directly applied to the mixed RF. In such a scheme, one would permute the SNPs that are used for the RF feature learning, whereas keeping the relationship between the random effect covariance matrix (kinship) and the phenotype intact. The latter is important to retain control for population structure, see, for example, ref. 65 . Alternatively, simulation-based approaches have been proposed for LMMs [57] , [58] . Provided that effects of independent noise and population structure can be correctly estimated from the data, these methods might help to further improve statistical power/runtime as compared with permutation-based approaches. Forest parameter settings In general, we aimed to keep parameter settings between RF and mixed RF as consistent and comparable as possible. Unless stated otherwise, we considered ensembles of 250 trees for both RF and mixed RF. Each tree was grown on a bootstrap sample (sampling with replacement) of full training set size. We considered a random subsample of 2/5 of all available predictors to determine the best split. However, if computational resources allow, fitting of this parameter (for example, via cross-validation) might be considered to further improve performance. Splitting of tree nodes was stopped if they contained less than five samples. Implementation of comparison partners With exception of the runtime experiments, we use our own mixed RF implementation to ‘implement’ a standard RF. This can straightforwardly be achieved by setting the covariance matrix Σ to the identity matrix, where the mixed RF is equivalent to a standard RF. The LASSO was used to optimize the following LM where X denotes full matrix of M genomic features (columns) for N individuals (rows), y is the N × 1 vector of phenotypic measurements and is iid Gaussian noise. The LASSO minimizes the L1-penalized mean squared error with respect to model weights β The LASSO implementation we considered was contained in the scikit-learn python package [62] . Therein, we set the optimization method to the (default) coordinate descent algorithm to find the most probable feature weights . The LMM LASSO model [17] is the conceptually straightforward extension to the LASSO model in equation (10), which also includes a random effect u to account for confounding where Here, the covariance Σ is identical to the covariance employed in the mixed RF and can be, if modelling of population structure is intended, estimated by the realized relationship matrix (RRM) [66] . Consequently, the updated error function now also includes contribution of the random effect For further details to inference in this model, we refer to ref. 17 . Again, we used scikit-learn as a basis to implement the LMM LASSO. To fit the LMM, we used a python-based implementation, which follows the derivation of fastLMM [2] . The standard LM is implemented in the same framework, setting Σ = I . LM-BLUP is a simple two-stage extension of the LM. In the first step, we estimate the effect of population structure computing the BLUP [36] based on the kinship matrix that is also used by our mixed RF and LMM LASSO. We subtract the estimated population effect from the phenotype and compute the univariate LM in the second stage on the residuals. RF-BLUP implements the analogoue BLUP-based correction for population effects and computes the standard RF on the residuals. Simulation study We used genetic features obtained in the form of SNPs from the study by Atwell et al . [35] . For each simulation experiment, we considered a random subset of 1,000 SNPs with a minor allele frequency (MAF) >0.1. In our basline setting (as indicated by the asterisk in Fig. 2 ) we simulate a total of 50 traits for 250 individuals as follows: three randomly chosen SNPs were considered as causal markers to simulate linear additive effects and further three pairs of SNPs were chosen to contribute epistatic effects where , and . Interaction effects were simulated by taking the component-wise binary product as indicated by the ‘int’ operator above. This corresponds to interactions between both minor alleles. In principle, mixed RF and RF are agnostic to the type of epistasis and hence, we did not consider other interactions (major–major, major–minor and so on). The resulting vector is multiplied by the simulated effect size β i . The polygenic effect u is a sample from a multivariate gaussian having the realized relationship matrix Σ [66] as covariance. Here, Σ is constructed from another subsample of 1,000 SNPs. Contributions of fixed genetic effect, polygenic effect and independent gaussian noise to the total trait variance are split into 0.375:0.5:0.125 adjusting and accordingly. To compare alternative methods in different genetic settings, we vary the relative number of additive and interaction terms (6:0–0:6, Fig. 2a ), the ratio of variance by population structure and independent noise (0.1–0.9, Fig. 2b ), the total number additive and interaction terms (1 interaction and 1 additive term–10 interaction and 10 addive terms, Fig. 2c ) and the relative contribution of independent noise (0.125–0.59, Supplementary Fig. 2d ) adjusting the simulation set-up (equation (15)) accordingly. Here we employ bootstrapping of half the number of samples for both RF and mixed RF. To obtain feature scores for we use the residual sums of squares (RFRSS) as described above. For both LASSO and LMM LASSO, we followed the procedure in ref. 17 and scored features by their order of inclusion. This approach avoids choosing a fixed regularization by successively lowering the shrinkage parameter λ until all variables are included into the model. To assess the importance of features for the univariate LMs (LM and LMM), we employ likelihood ratio tests [67] . To correct for confounding in this experiments on semi-synthetic A. thaliana data, we employ the realized relationship matrix that was used to simulate population structure. Mouse eQTL-mapping experiment We considered gene expression measured in hippocampus tissue of 468 heterogeneous stock (HS) mice where genotype information was given in the form of 12,545 genome-wide SNPs [39] . From a total of 19,892 expression traits, we selected the top 10 percentile ranked by variance (1,989). From these, 373 could be associated to at least one Reactome pathway. To establish an association between SNP and genes in the pathway database, we considered all (ENSEMBL) annotated genes within a 500-kb window around the SNP. An association between SNP x i and gene j was considered as ‘Reactome consistent’ if at least one of the genes linked to SNP x i had a pathway in common with gene j . We did not consider links that were induced by cis effects according to our 500-kb distance threshold. We further excluded expression traits that were linked to less than 10 or more than 1,000 SNPs. For each method, we ranked SNPs by their QTL scores for all of the 300 remaining traits, resulting in a single ranking of all 300*12,545 SNP–trait pairs. Each point on a curve as shown in Fig. 3 reports the number of Reactome-consistent associations that are recovered, normalized by the number of consistent associations expected from a random SNP ranking. For scoring eQTLs, we use the same feature importance measures as in our simulation study, with the exception of LASSO and LMM LASSO. Here, we found that the recently proposed stability selection [54] is more robust (see also discussion in ref. 17 ). The rationale behind this is, that in contrast to our simulation study, we aggregate over a large number of traits each having a different number of informative genetic features (if any). Just using the ranks from the inclusion path in a single LASSO run would be inapproriate, because that would not account for the variable number of informative markers for each trait. We implemented stability selection as follows. For each of the expression traits, we randomly sampled 90% of the data without replacement and learn the LASSO/LMM LASSO model such that it includes 20 features (adjusting the shrinkage parameter λ accordingly). We repeated this random sampling and learning 1,000 times, reporting the fraction of times a feature was selected as an importance score. To estimate the kinship for mixed RF and LMM LASSO, we first used a simple linear association test to rank all SNPs by their log odds ratio [67] and subsequently selected the top 1,000 genetic features to build the RRM. This ranking avoids inclusion of features that explain little of the overall variance (see also ref. 33 for a discussion on selecting subsets of features for building RRMs). Prediction experiment of global mouse phenotypes We selected a total of 124 phenotypes (ranging from biochemical to behavioural traits) measured in a total of 1,904 mouse HS individuals [49] , [68] (see Supplementary Data 1 for a full list). Parts of the same cohort were used for eQTL mapping, thus we have the same genotype information of 12,545 genome-wide SNPs. For prediction of the mouse phenotypes, we used ensembles of 100 trees. For learning each mixed RF regression tree, we randomly sampled without replacement half the training set. This leaves the remaining half of the training data to adjust the depth of the trees. For the RF we use subsampling with replacement, since the used python package [62] does not provide subsampling without replacement. For the task of phenotype prediction, the available sample size was much larger (as compared with the eQTL-mapping experiment before) and hence, we used all 12,545 genetic features to estimate the population structure using the RRM as before. Alternatively, a rank-based feature filtering as for the eQTL study above could have been considered, which may improve the prediction performance of methods with random effect terms. The shrinkage parameter λ required for LASSO and LMM LASSO was selected using a nested fivefold randomized cross-validation on a fine grid. Application to the NFBC data We analysed data from the NFBC1966 cohort [50] , considering four blood lipid phenotypes (C-reactive protein, triglycerides, low-density lipoprotein and high-density lipoprotein cholesterol levels) for a total of 5,256 unrelated individuals. Following the approach taken in ref. 52 , we quantile-normalized each trait to follow a unit variance normal distribution. We used genetic features (SNPs) for a total of 328,517 variants with a MAF of at least 1%. We used the same set of SNPs to estimate the realized relationship matrix used to correct for the effects of population structure. For each of the four lipid traits, we learned a mixed RF having 250 trees. To avoid imbalanced trees, we grew trees to a maximal depth of 12 (≈log 2 (5256)). We used a random subsample of half of the individuals (drawn without replacement) to learn each regressor. Here, 60% of the genetic features were randomly subsampled to perform each split. We rank all genetic loci (SNPs) by their score and reported the top 40 hits sorted by chromosome and position (see Supplementary Data 2 ). Runtime and computational complexity In general, the runtime of all mapping methods (LMM, LMM LASSO, standard RF and the mixed RF) scales linearly with the number of markers. This is a very important feature, since the typical number of markers drastically exceeds the number of individuals. However, the methods differ with respect to their dependency on the number of individuals. Methods correcting for population structure (LMM, LMM LASSO and the mixed RF) scale cubic with the number of individuals (due to the singular value decomposition of the realized relationship matrix). For comparison, the standard RF only scales with a complexity of in the number of individuals. The amount of memory required by mixed RF is quadratic in the number of samples (storing of the realized relationship matrix Σ ) and otherwise similar to that of the standard RF (that is, linear in the number of genetic features). Optimizing regression tree implementations is a complex task. At the time of writing this paper, our method is primarily tuned for handling many genetic features (that is, scenarios where M ≫ N ). Significant speedups are to be expected if one uses a low-rank approximation of the relationship matrix ( Σ ), which allows to apply the same computational tricks as introduced in ref. 2 . Also, adjusting the model complexity (tree depths) for feature selection tasks may be considered. Consequently, less splits are needed thereby decreasing the runtime. For mouse phenotype prediction, our methods run on data with 1,940 individuals for each of which we have 12,545 genetic features (SNPs). For a given phenotype, the current mixed RF implementation takes on average about 1,402 s (with an empirical s.d. of 1,096 s) for a single fold within the fivefold cross-validation. The high variations in runtime are due to individual depths up to which forests are grown. Thus, runtimes of 5–40 min are to be expected if one intends to train a single model on a data set of similar size. In comparison, RF takes 103 s (s.d. 36 s), that is, typically 1.5–2.5 min for a single trait. For the remaining methods, we measured the following runtimes: LMM LASSO 521 s (s.d. 177 s), LASSO 598 s (s.d. 148 s) and BLUP 12 s (s.d. 2 s). In the case of our mixed RF implementation, the memory requirement never exceeded two gigabyte of RAM. All experiments (including the application of mixed RF to the Norhtern Finnland Birth Cohort) were executed on individual Intel Xeon E5-2670 2.60 GHz processors. Software availability The mixed RF is part of the LIMIX [69] software package, which is freely available on https://github.com/PMBio/limix . How to cite this article: Stephan, J. et al . A random forest approach to capture genetic effects in the presence of population structure. Nat. Commun. 6:7432 doi: 10.1038/ncomms8432 (2015).